The solute carrier SLC9C1 is a Na+/H+-exchanger gated by an S4-type voltage-sensor and cyclic-nucleotide binding Voltage-sensing (VSD) and cyclic nucleotide-binding domains (CNBD) gate ion channels for rapid electrical signaling. By contrast, solute carriers (SLCs) that passively redistribute substrates are gated by their substrates themselves. Here, we study the orphan sperm-specific solute carriers SLC9C1 that feature a unique tripartite structure: an exchanger domain, a VSD, and a CNBD. Voltage-clamp fluorimetry shows that SLC9C1 is a genuine Na + /H + exchanger gated by voltage. The cellular messenger cAMP shifts the voltage range of activation. Mutations in the transport domain, the VSD, or the CNBD strongly affect Na + /H + exchange, voltage gating, or cAMP sensitivity, respectively. Our results establish SLC9C1 as a phylogenetic chimaera that combines the ion-exchange mechanism of solute carriers with the gating mechanism of ion channels. Classic SLCs slowly readjust changes in the intra- and extracellular milieu, whereas voltage gating endows the Na + /H + exchanger with the ability to produce a rapid pH response that enables downstream signaling events. Solute carriers (SLC), only second to GPCRs, form one of the largest gene families in vertebrates, comprising about 450 members in the human genome. Yet, compared to other gene families, SLCs are understudied and many isoforms represent orphan proteins, highlighting our ignorance [1] . A case in point is the subfamily SLC9C1, also referred to as sNHE. SLC9C1 has been suspected to serve as Na + /H + exchanger that controls intracellular pH (pH i ) in mammalian sperm [2] . Changes in pH i are key to sperm signaling [3] , [4] , [5] , [6] , [7] , [8] , [9] , [10] , [11] , but it is not known if SLC9C1 indeed promotes Na + /H + exchange, how its activity is controlled, and whether it contributes to pH i regulation. Disrupting the mouse slc9c1 gene renders sperm immotile and male mice infertile [2] , [12] , demonstrating that SLC9C1 is required for sperm function and fertilization in mammals. However, the pH i of SLC9C1 −/− sperm is not altered [2] , and a clear-cut conclusion is compounded by the unexpected observation that cAMP synthesis is impaired in SLC9C1 −/− sperm and that the motility defect can be rescued by cAMP [12] , [13] . These observations suggest that the prime defect of SLC9C1 −/− sperm might be in cAMP—rather than pH i signaling. Finally, mouse SLC9C1 is non-functional in heterologous systems and attempts to study SLC9C1-mediated Na + /H + exchange by pH i fluorimetry in mouse sperm were unsuccessful [2] . Thus, the function of SLC9C1 as a Na + /H + exchanger and its role in pH i regulation of mammalian sperm is left in limbo. On a different yet related note, in sea urchin sperm, chemoattractants stimulate a rapid rise of pH i [9] , [14] , [15] , [16] , [17] , [18] , [19] , [20] , which serves as a switch to activate the pH-sensitive CatSper Ca 2+ channel that controls chemotaxis [9] . The molecule underlying this alkalinization is not known. However, a Na + /H + exchange mechanism was described that is activated by hyperpolarization rather than by changes in the extracellular pH or Na + concentrations [14] , [15] , [17] . Ever since its discovery, the activation of Na + /H + exchange by voltage and the underlying mechanism and molecules have remained unexplained. We report here final success in solving these fundamental and long-standing questions. We demonstrate that the Strongylocentrotus purpuratus homolog ( Sp SLC9C1) exists in sperm and represents a genuine Na + /H + antiporter. Unlike solute carriers, Na + /H + exchange by Sp SLC9C1 is gated by voltage via a voltage-sensing domain (VSD) and directly modulated by cAMP via a cyclic nucleotide-binding domain (CNBD). Thus, we deorphanize the SLC9C1 family and identify Na + /H + exchange as a target for cAMP signaling and a mechanism of adaptive interaction between pH i and cAMP. On a broader perspective, our results now enable future studies of the commonalities and differences of voltage sensing and cAMP modulation between ion channels and a solute carrier and, thereby, gain insight into the evolution of gating mechanisms. Overall protein topology of SLC9C1 Sperm-specific Na + /H + exchangers share with SLC9 family members the exchanger domain that carries substrates across membranes. In addition, SLC9C1 holds a putative voltage-sensing domain (VSD) and a putative cyclic nucleotide-binding domain (CNBD) that are absent in other SLC9 members (Fig. 1a ). The exchange domain of Sp SLC9C1 is predicted to encompass 14 transmembrane segments (TM), whereas bacterial and archaeal Na + /H + exchangers feature 12 and 13 TMs, respectively [21] , [22] , [23] . A sequence alignment illustrates that Sp SLC9C1 carries an additional TM at the N-terminal end (Fig. 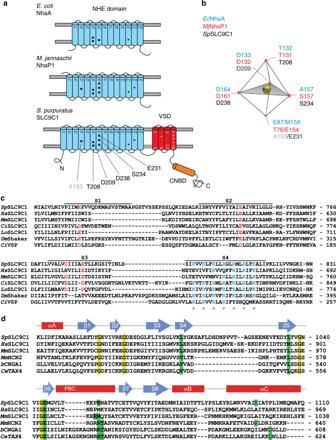Fig. 1 Structural features ofSpSLC9C1.aTransmembrane topology ofEscherichia coliNhaA (EcNhaA),Methanocaldococcus jannaschiiNhaP1 (MjNhaP1), and sea urchinStrongylocentrotus purpuratusSLC9C1 (SpSLC9C1); VSD voltage-sensing domain, CNBD cyclic nucleotide-binding domain. Amino acids that may participate in Na+coordination are highlighted (black dots). Asterisks indicate conserved Arg residues that are relevant for Na+/H+antiport; Arg320 and Arg347 inMjNhaP1; Arg399 and Arg431 inSpSLC9C1. An Arg is substituted by Lys300 inEcNhaA.bScheme of the trigonal bi-pyramidal structure of the Na+coordination site fromMjNhaP1. Numbers refer to the respective amino-acid residues inE. coli(blue),M. jannaschii(red), andS. purpuratus(black).cSequence comparison of the VSD from several SLC9C1 members with the canonical VSD ofDrosophilaShaker K+channel (DmShaker) andCiona intestinalisvoltage-sensor-containing-phosphatase (CiVSP).S. purpuratus(SpSLC9C1),H. sapiens(HsSLC9C1),M. musculus(MmSLC9C1),C. intestinalis(CiSLC9C1), and spotted garL. oculatus(LoSLC9C1). Voltage sensors carry conserved positively charged residues in S4 (blue) and conserved negatively charged amino acids in S1–S3 (red).dCyclic nucleotide-binding domains from sea urchin (SpSLC9C1), human (HsSLC9C1) and mouse (MmSLC9C1) SLC9C1, mouse HCN channelMmHCN2, bovine CNG channelbCNGA1, andC. elegansCNG channel (CeTAX4). The CNBD comprises three α-helices (αA, αB, and αC), eight β-strands (β1–β8), and a phosphate-binding cassette (PBC). Highlighted key residues are the purine-binding residues Val and Leu (β4 and β5), the ribofuranose-binding residues Gly/Glu (β6), the phosphate-binding residues Arg/Thr, and the purine-binding Arg in αC ofMmHCN2 1a and Supplementary Figure 1 ). The Na + -binding site in archaeal SLC9 forms a trigonal bipyramid [22] , [23] . In Methanocaldococcus jannaschii NhaP1, two carboxyl groups (D132 and D161) and a hydroxyl group (S157) form a triangle around Na + ; the main-chain carbonyl of T131 is positioned at one bipyramid tip and T76/E154 at the other tip (Fig. 1b ). All but one of the important Na + -coordinating residues are conserved in Sp SLC9C1, including an Asn/Asp motif (Asn237/Asp238) that is diagnostic for electroneutral exchangers [24] (Fig. 1a, b ). Residues occupying the (T76/E154) pyramid tip are less conserved, even among archaeal SLCs. Furthermore, two Arg residues in TMs 12 and 13 that are functionally important in other Na + /H + exchangers are conserved in Sp SLC9C1 (Fig. 1a and Supplementary Figure 1 ). Fig. 1 Structural features of Sp SLC9C1. a Transmembrane topology of Escherichia coli NhaA ( Ec NhaA), Methanocaldococcus jannaschii NhaP1 ( Mj NhaP1), and sea urchin Strongylocentrotus purpuratus SLC9C1 ( Sp SLC9C1); VSD voltage-sensing domain, CNBD cyclic nucleotide-binding domain. Amino acids that may participate in Na + coordination are highlighted (black dots). Asterisks indicate conserved Arg residues that are relevant for Na + /H + antiport; Arg320 and Arg347 in Mj NhaP1; Arg399 and Arg431 in Sp SLC9C1. An Arg is substituted by Lys300 in Ec NhaA. b Scheme of the trigonal bi-pyramidal structure of the Na + coordination site from Mj NhaP1. Numbers refer to the respective amino-acid residues in E. coli (blue), M. jannaschii (red), and S. purpuratus (black). c Sequence comparison of the VSD from several SLC9C1 members with the canonical VSD of Drosophila Shaker K + channel ( Dm Shaker) and Ciona intestinalis voltage-sensor-containing-phosphatase ( Ci VSP). S. purpuratus ( Sp SLC9C1), H. sapiens ( Hs SLC9C1), M. musculus ( Mm SLC9C1), C. intestinalis ( Ci SLC9C1), and spotted gar L. oculatus ( Lo SLC9C1). Voltage sensors carry conserved positively charged residues in S4 (blue) and conserved negatively charged amino acids in S1–S3 (red). d Cyclic nucleotide-binding domains from sea urchin ( Sp SLC9C1), human ( Hs SLC9C1) and mouse ( Mm SLC9C1) SLC9C1, mouse HCN channel Mm HCN2, bovine CNG channel b CNGA1, and C. elegans CNG channel ( Ce TAX4). The CNBD comprises three α-helices (αA, αB, and αC), eight β-strands (β1–β8), and a phosphate-binding cassette (PBC). Highlighted key residues are the purine-binding residues Val and Leu (β4 and β5), the ribofuranose-binding residues Gly/Glu (β6), the phosphate-binding residues Arg/Thr, and the purine-binding Arg in αC of Mm HCN2 Full size image The full-fledged VSD (four transmembrane domains S1–S4) of Sp SLC9C1 carries seven conserved Arg or Lys residues in the S4 motif and four conserved Glu or Asp residues in S1–S3 (Fig. 1c ). Finally, the CNBD features the hallmarks of a cyclic nucleotide-binding fold: three α-helices (αA, αB, and αC), eight β-strands (β1–β8), and a phosphate-binding cassette (PBC) (Fig. 1d ). Key residues that interact with cyclic nucleotides are conserved, including the purine-binding residues Val and Leu (β4 and β5), the ribofuranose-binding residues Gly/Glu (β6), the phosphate-binding Arg between β6 and β7, and the purine-binding residues Arg/Lys in αC [25] , [26] . The presence of exchanger, VSD, and CNBD domains suggests that SLC9C1 promotes Na + /H + exchange controlled by voltage and cyclic nucleotides. We studied by heterologous expression of Sp SLC9C1 its voltage sensitivity, Na + /H + exchange activity, and regulation by cyclic nucleotides. The voltage-sensing domain produces gating currents For electrophysiological experiments, we used CHO cells stably expressing HA-tagged Sp SLC9C1. 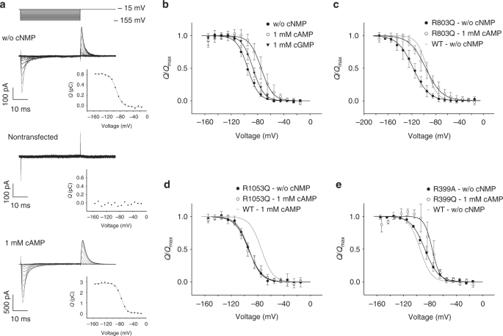Fig. 2 Gating currents ofSpSLC9C1. Voltage protocol, gating currents, and charge–voltage (Q/V) relation. The solid curve in theQ/Vrelations (insets) represents a Boltzmann fit.aUpper: wtSpSLC9C1 without cNMP (V1/2= −91.4 mV, slopes=9.2 mV). Middle: non-transfected CHO cells. Lower: wtSpSLC9C1, 1 mM cAMP in the pipette solution (V1/2= −75.4 mV,s=8.2 mV).bQ/Qmaxvs.Vmrelation. Mean ± SD (n= number of experiments) ofV1/2and slopeswas determined by a Boltzmann fit (w/o cNMP: −94.7 ± 2.9 mV,s= 8.5 ± 0.8 mV,qg= 3.1e0,n= 6; cAMP: −74.4 ± 6.4 mV,s= 8.8 ± 1.9 mV,qg= 2.9e0,n= 7; cGMP: −86.9 ± 3.0 mV,s= 8.3 ± 1.0 mV,qg= 3.1e0,n= 7).cReplacing Arg803 in S4 by Gln (R803Q) shiftedV1/2by −24 mV andsby 5 mV (V1/2= −117.9 ± 7.1 mV,s= 13.0 ± 1.1 mV,qg= 2.0e0,n= 7). This mutation did not affectV1/2modulation by 1 mM cAMP (V1/2= −96.8 ± 6.6 mV,s= 13.5 ± 2.6 mV,qg= 1.9e0,n= 6). Gray line: voltage dependence of wtSpSLC9C1 without cNMP.dReplacing Arg1053 in the CNBD by Gln (R1053Q) does not affectV1/2without cNMP (−93.4 ± 1.7 mV,s= 9.4 ± 2.0 mV,qg= 2.8e0,n= 6), but strongly reducedV1/2shift by cAMP (V1/2= −93.9 ± 4.2 mV,s= 10.3 ± 1.0 mV,qg= 2.5e0,n= 5). Gray line: voltage dependence of wtSpSLC9C1 with cNMP.eIn the NHE-domain mutant (R399A), Na+/H+exchange is abolished (Fig.5), but not gating currents (Supplementary Figure4).V1/2in the absence (−87.3 ± 2.8 mV,s= 10.4 ± 1.8 mV,qg= 2.5e0,n= 3) and presence of cAMP (−76.5 ± 9.6 mV,s= 6.0 ± 0.8 mV,qg= 4.3e0,n= 5). Gray line: voltage dependence of wtSpSLC9C1 without cNMP An anti-HA antibody stained sheets of plasma membrane (Supplementary Figure 2 ), showing that Sp SLC9C1 reaches the cell membrane. We tested by whole-cell patch-clamping whether the VSD is functional and displays charge movements during voltage steps. In fact, several different ion channels, e.g., CNG channels, carry a VSD, yet are not gated by voltage and are not voltage-dependent. In voltage-activated ion channels, the movement of charged amino acids in S4 during activation produces so-called gating currents [27] . Brief voltage pulses (−15 to −155 mV) evoked transient negative and positive gating currents at the onset and termination of the voltage pulse, respectively (Fig. 2a ). In control cells, voltage steps did not evoke gating currents (Fig. 2a ). A fit of the Boltzmann function to the integrated off-gating currents yielded a voltage of half-maximal activation ( V ½ ) and slope factor ( s ) of −94.7 ± 2.9 and 8.5 ± 0.8 mV, respectively, corresponding to a gating charge q g of 3.1 e o (Fig. 2a, b and Table 1 ). In conclusion, the VSD in Sp SLC9C1 is functional. Fig. 2 Gating currents of Sp SLC9C1. Voltage protocol, gating currents, and charge–voltage ( Q / V ) relation. The solid curve in the Q / V relations (insets) represents a Boltzmann fit. a Upper: wt Sp SLC9C1 without cNMP ( V 1/2 = −91.4 mV, slope s = 9.2 mV). Middle: non-transfected CHO cells. Lower: wt Sp SLC9C1, 1 mM cAMP in the pipette solution ( V 1/2 = −75.4 mV, s = 8.2 mV). b Q / Q max vs. V m relation. Mean ± SD ( n = number of experiments) of V 1/2 and slope s was determined by a Boltzmann fit (w/o cNMP: −94.7 ± 2.9 mV, s = 8.5 ± 0.8 mV, q g = 3.1 e 0 , n = 6; cAMP: −74.4 ± 6.4 mV, s = 8.8 ± 1.9 mV, q g = 2.9 e 0 , n = 7; cGMP: −86.9 ± 3.0 mV, s = 8.3 ± 1.0 mV, q g = 3.1 e 0 , n = 7). c Replacing Arg803 in S4 by Gln (R803Q) shifted V 1/2 by −24 mV and s by 5 mV ( V 1/2 = −117.9 ± 7.1 mV, s = 13.0 ± 1.1 mV, q g = 2.0 e 0 , n = 7). This mutation did not affect V 1/2 modulation by 1 mM cAMP ( V 1/2 = −96.8 ± 6.6 mV, s = 13.5 ± 2.6 mV, q g = 1.9 e 0 , n = 6). Gray line: voltage dependence of wt Sp SLC9C1 without cNMP. d Replacing Arg1053 in the CNBD by Gln (R1053Q) does not affect V 1/2 without cNMP (−93.4 ± 1.7 mV, s = 9.4 ± 2.0 mV, q g = 2.8 e 0 , n = 6), but strongly reduced V 1/2 shift by cAMP ( V 1/2 = −93.9 ± 4.2 mV, s = 10.3 ± 1.0 mV, q g = 2.5 e 0 , n = 5). Gray line: voltage dependence of wt Sp SLC9C1 with cNMP. e In the NHE-domain mutant (R399A), Na + /H + exchange is abolished (Fig. 5 ), but not gating currents (Supplementary Figure 4 ). 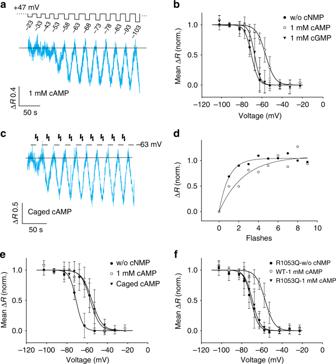Fig. 4 Modulation ofSpSLC9C1 activity by cAMP.aAction of 1 mM cAMP in the pipette solution on the voltage dependence ofSpSLC9C1 (V1/2= −53.4 mV). ([Na+]o0 mM; [Na+]i14 mM; pHi= 7.2; pHo= 7.4).bNormalized ΔRvalues were plotted againstVmto yield theV1/2values by a fit with the Boltzmann equation (w/o cNMP:V1/2= −70.9 ± 2.5 mV,s= 3.3 ± 0.9 mV,n= 7; cAMP:V1/2= −56.8 ± 2.7 mV,s=4.6 ± 1.5 mV,n= 7; cGMP:V1/2= −67.8 ± 5.4 mV,s=2.8 ± 1.0 mV,n= 9).cFlash photolysis of caged cAMP enhancedSpSLC9C1 activity at a holding voltage of −63 mV and saturated after 3–4 flashes, same conditions as ina.dNormalized ΔRvalues were plotted against the number of flashes. Black circles show values fromc. Decreasing the light energy of the flash, saturation ofSpSLC9C1 activity required 5–6 flashes (white circles).eThe shift ofV1/2andsvalues evoked by flash photolysis were similar to those using cAMP in the pipette (black triangles:V1/2= −55.3 ± 5.1 mV,s=5.0 ± 0.6 mV,n= 3; for comparison: w/o cNMP (black circles) and 1 mM cAMP (white circles).fReplacing the Arg1053 in the CNBD by Gln (R1053Q) maintained a wild-type-likeV1/2in the absence of cNMP (−70.8 ± 4.8 mV,s= 3.6 ± 1.1 mV,n= 5), but strongly reduced theV1/2shift by cAMP (−69.5 ± 3.8 mV,s= 3.9 ± 1.2 mV,n= 6). Mean values are summarized in Table1 V 1/2 in the absence (−87.3 ± 2.8 mV, s = 10.4 ± 1.8 mV, q g = 2.5 e 0 , n = 3) and presence of cAMP (−76.5 ± 9.6 mV, s = 6.0 ± 0.8 mV, q g = 4.3 e 0 , n = 5). Gray line: voltage dependence of wt Sp SLC9C1 without cNMP Full size image Table 1 Summary of activation properties of Sp SLC9C1 from gating currents and voltage-clamp fluorimetry Full size table In voltage-gated K + channels, substituting Arg residues in the S4 motif for neutral residues shifts V ½ to more negative values [28] , [29] , [30] , [31] , [32] . Replacing the third Arg residue in the S4 segment of Sp SLC9C1 by Gln (R803Q) shifted the V ½ of gating-current activation by −24 to −117.9 ± 7.1 mV (Fig. 2c and Supplementary Figure 4a ); concomitantly, the number of gating charges was lowered to 2.0 e o (Fig. 2c and Table 1 ). Arg803 apparently contributes one equivalent gating charge, indicating that it may cross the entire transmembrane electric field, similar to the homologous Arg368 in Shaker K + channels [32] . Sp SLC9C1 mediates voltage-gated Na + /H + exchange No currents other than gating currents were observed, indicating that Na + /H + exchange is electroneutral. We tested Na + /H + exchange activity of Sp SLC9C1 in the whole-cell configuration by voltage-clamp fluorimetry, using the pH indicator BCECF. For inwardly directed Na + gradients, stepping V m from −40 to −100 mV enhanced the BCECF fluorescence ratio R ( F 480 / F 440 ), indicating intracellular alkalinization (Fig. 3a ). After the voltage was stepped back, exchange activity stopped and pH i slowly returned to baseline (Fig. 3a ). In non-transfected cells, this voltage protocol did not change pH i , showing that potential endogenous Na + /H + exchangers do not operate under these conditions (Fig. 3a ). Additional controls ascertain that the changes in pH i result from Na + /H + exchange of Sp SLC9C1: first, when extracellular Na + was substituted for NMDG, i.e., when the Na + gradient was reversed, the fluorescence ratio decreased upon hyperpolarization, reflecting intracellular acidification (Fig. 3b ). Second, when both pH and [Na + ] are symmetric across the membrane, stepping V m to −100 mV did not change pH i (Fig. 3c ). The suppression was reversible: when the Na + gradient was restored, hyperpolarization again evoked alkalinization (Fig. 3c ). 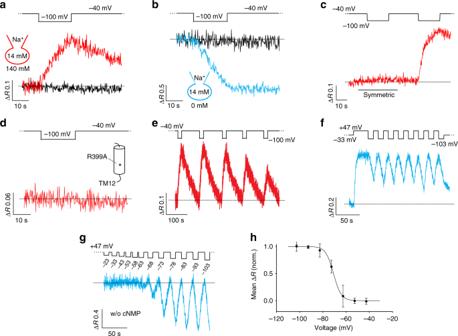Furthermore, we compared the pH i buffer capacity and resting pH i (pH rest ) of control CHO- and CHO- Sp SLC9C1 cells using the pH i pseudo-null-point method [9] , [33] , [34] , [35] , [36] . Fig. 3 Voltage-clamp pHifluorimetry ofSpSLC9C1 activity.aAlkalinization induced by a 20 s step hyperpolarization to −100 mV using an inwardly directed Na+gradient ([Na+]i14 mM; [Na+]o140 mM; pHi= 7.2; pHo= 7.4, forward mode, red). No pHichange occurred in non-transfected CHO cells (black).bAcidification induced by a 20 s step hyperpolarization to −100 mV using an outwardly directed Na+gradient ([Na+]i14 mM; [Na+]o0 mM; pHi= 7.2; pHo= 7.4, reverse-mode, blue).cPerfusion with symmetric solutions (black line) abolished the net Na+/H+exchange due to a lacking gradient (pHi= pHo= 7.2, [Na]i= [Na]o= 14 mM). Voltage induced net Na+/H+exchange was restored when the cell was perfused with 140 mM Na+(pHo= 7.4).dWhen Arg399 in T12 of the exchanger domain is replaced by Ala (R399A), Na+/H+exchange was abolished.epHiresponses to repetitive voltage steps from −40 to −100 mV in a CHO-SpSLC9C1 cell. Dotted line indicates resting pHi. ([Na+]i14 mM; [Na+]o140 mM; pHi= 7.2; pHo= 7.4).fRepetitive stimulation ofSpSLC9C1 activity (reverse mode) in CHO cells that co-express the H+-selective channel Hv1. Cells quickly recovered from acidification by activation of Hv1 at +47 mV. ([Na+]i14 mM; [Na+]o0 mM; pHi= 7.2; pHo= 7.4).gVoltage dependence ofSpSLC9C1 activation was determined by steppingVmbetween −23 and −103 mV to +47 mV (V1/2= −70.4 mV; [Na+]i14 mM; [Na+]o0 mM; pHi= 7.2; pHo= 7.4).hNormalized ΔRvalues were plotted againstVmto yield theV1/2values by a fit with the Boltzmann equation (V1/2= −70.9 ± 2.5 mV,s= 3.3 ± 0.9 mV,n= 7). Mean values are summarized in Table1 The pH i changes imposed by the respective pH i pseudo-null-point solutions were similar in control CHO- and CHO- Sp SLC9C1 cells (Supplementary Figure 3a, b ), showing that expression of Sp SLC9C1 per se neither affects the pH i and buffering capacity of cells nor the kinetics and magnitude of the pH-indicator response. Fig. 3 Voltage-clamp pH i fluorimetry of Sp SLC9C1 activity. a Alkalinization induced by a 20 s step hyperpolarization to −100 mV using an inwardly directed Na + gradient ([Na + ] i 14 mM; [Na + ] o 140 mM; pH i = 7.2; pH o = 7.4, forward mode, red). No pH i change occurred in non-transfected CHO cells (black). b Acidification induced by a 20 s step hyperpolarization to −100 mV using an outwardly directed Na + gradient ([Na + ] i 14 mM; [Na + ] o 0 mM; pH i = 7.2; pH o = 7.4, reverse-mode, blue). c Perfusion with symmetric solutions (black line) abolished the net Na + /H + exchange due to a lacking gradient (pH i = pH o = 7.2, [Na] i = [Na] o = 14 mM). Voltage induced net Na + /H + exchange was restored when the cell was perfused with 140 mM Na + (pH o = 7.4). d When Arg399 in T12 of the exchanger domain is replaced by Ala (R399A), Na + /H + exchange was abolished. e pH i responses to repetitive voltage steps from −40 to −100 mV in a CHO- Sp SLC9C1 cell. Dotted line indicates resting pH i . ([Na + ] i 14 mM; [Na + ] o 140 mM; pH i = 7.2; pH o = 7.4). f Repetitive stimulation of Sp SLC9C1 activity (reverse mode) in CHO cells that co-express the H + -selective channel Hv1. Cells quickly recovered from acidification by activation of Hv1 at +47 mV. ([Na + ] i 14 mM; [Na + ] o 0 mM; pH i = 7.2; pH o = 7.4). g Voltage dependence of Sp SLC9C1 activation was determined by stepping V m between −23 and −103 mV to +47 mV ( V 1/2 = −70.4 mV; [Na + ] i 14 mM; [Na + ] o 0 mM; pH i = 7.2; pH o = 7.4). h Normalized Δ R values were plotted against V m to yield the V 1/2 values by a fit with the Boltzmann equation ( V 1/2 = −70.9 ± 2.5 mV, s = 3.3 ± 0.9 mV, n = 7). Mean values are summarized in Table 1 Full size image The NhaP1 of M. jannaschii harbors two essential Arg residues in transmembrane segments T11 (R320) and T12 (R347) (Supplementary Figure 1 ) [24] . When these residues in NhaP1 are mutated to Ala, the exchange activity is abolished (R320A) or severely impaired (R347A) [24] . We replaced in Sp SLC9C1 the Arg residue, which is homologous to R320, by an Ala residue (R399A in TM12 (Supplementary Figure 1 )). The R399A mutant produced gating currents with a V 1/2 and steepness s similar to those of the wild-type protein (Fig. 2e and Supplementary Figure 4b ). However, Na + /H + exchange activity was abolished in the R399A mutant (Fig. 3d ). This result shows that in the R399A mutant transport activity of the exchanger domain is abolished without affecting the gating mechanism. In conclusion, Sp SLC9C1 is a genuine Na + /H + exchanger that, like other ion exchangers, can operate in the forward and reverse mode. Voltage dependence of exchange activity We determined the voltage dependence of Sp SLC9C1 by recording Na + /H + exchange activity at different voltages from one and the same cell. However, after stepping the voltage back to V hold , the pH i returned only slowly to resting levels (Fig. 3a, b ). Moreover, pH i signals started to run down during repetitive Sp SLC9C1 activation, which prevented recording a complete voltage-response relation under stable conditions (Fig. 3e ). To overcome these limitations, we co-expressed Sp SLC9C1 with the proton channel Hv1 and recorded Sp SLC9C1 activity in the reverse mode. The rationale underlying this strategy was: in the reverse mode, Sp SLC9C1 activity acidifies the cell (Fig. 3b ); subsequently, opening of Hv1 channels causes H + efflux and restores the original pH i . This prediction is borne out by experiments; upon hyperpolarization, Sp SLC9C1 activity acidifies the cell, and activation of H + outward currents via Hv1 by a subsequent depolarization [37] hastens the recovery from acidification (Fig. 3f ). Because the operative voltage regimes of Hv1 and Sp SLC9C1 do not overlap, H + efflux via Hv1 does not interfere with H + import via Sp SLC9C1. Sp SLC9C1 is activated at V m < −50 mV, whereas for the pH gradients used here, Hv1 opens at V m ≥ 0 mV [38] . Furthermore, Hv1 only supports H + outward currents [38] . In CHO cells expressing only Hv1, stepping V m from values between −23 and −113 mV to +47 mV produced a rapid Hv1-mediated increase of pH i , whereas stepping voltage from +47 mV to negative values did not change pH i (Supplementary Figure 3c ). When Sp SLC9C1 and Hv1 were co-expressed, the voltage protocol started with Hv1 activation to produce an initial alkalinization. This protocol provides a larger dynamic range of the BCECF dye, and the initial pH i value from which the Sp SLC9C1-mediated acidification started was always identical. In addition, this activation protocol ensures that the voltage dependence of Hv1 does not overlap with that of the Sp SLC9C1 protein, because alkalinisation shifts the voltage dependence of Hv1 activation to more positive voltages. Repetitive Hv1 activation (for 10 s at about +50 mV) followed by Sp SLC9C1 activation (for 10 s at about −100 mV) produced sawtooth-like cycles of alkalinization and acidification that were highly reproducible (Fig. 3f ). Therefore, Sp SLC9C1 activity at different voltages can be compared quantitatively. The voltage dependence of pH i responses was determined by stepping V m from a holding potential of +47 mV to values from −23 to −103 mV (Fig. 3g ). A Boltzmann function fitted to the initial slope Δ R s −1 vs. V m yielded a mean V ½ of −70.9 ± 2.5 mV and slope factor s = 3.3 ± 0.9 mV (Fig. 3h and Table 1 ). The pH i responses were similar when the V m protocol was reversed (Supplementary Figure 3d ). We tested several generic inhibitors of Na + /H + exchangers present in somatic cells [39] . 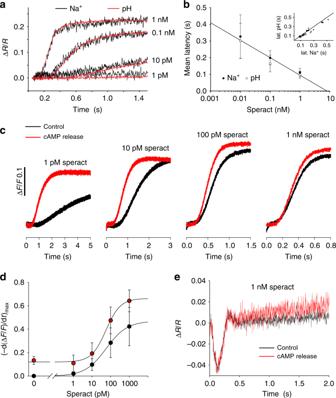Fig. 5 Sodium and proton fluxes inS. pupuratussperm.aSperact-induced changes in fluorescence ratio (ΔR/R) indicating Na+influx (ANG2, black) or proton efflux (pHi) (BCECF, red); signals were scaled and superimposed. Speract concentrations are shown on the right.bMean latency ± SD (n= 7) of pHiand Na+signal plotted vs. speract concentration. Inset: latency of pHiand Na+signal at different speract concentrations (10 pM black circles; 100 pM white circles; and 1 nM triangles). The line represents the identity function (n= 7).cSperact-induced alkalinization monitored by pHrodo Red fluorescence in the absence (black trace) or presence (red trace) of release of cAMP from DEACM-caged cAMP with a continuously pulsing UV-LED. UV light was applied during the entire recording time.dThe maximal slope of the pHrodo Red time course was plotted vs. speract concentration in the absence (black) and presence (red) of cAMP released from DEACM-caged cAMP (n= 3).eVoltage recordings during speract stimulation (1 nM) in the absence (black) or presence (red) of cAMP released from DEACM-caged cAMP None of these drugs affected the voltage-gated Na + /H + exchange activity or voltage dependence of Sp SLC9C1 activation (Supplementary Figure 5 a, b, c, d), most likely because the sequence motifs and regions to which these NHE inhibitors bind [40] are either lacking or different in Sp SLC9C1. The insensitivity of Sp SLC9C1 to amiloride provided an opportunity to confirm that endogenous Na + /H + exchangers in CHO cells are silent under our measuring conditions. 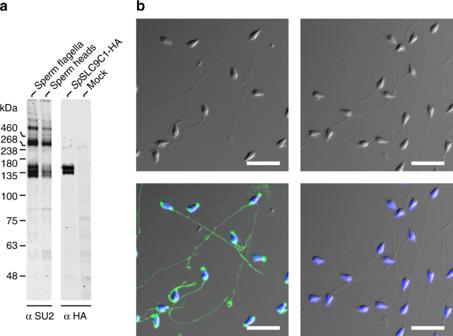Fig. 6 Analysis ofSpSLC9C1 expression in sea urchin sperm.aRepresentative western blot using protein lysates from flagella and heads ofS. purpuratussperm, from CHO cells heterologously expressing HA-taggedSpSLC9C1 (SpSLC9C1-HA), and from non-transfected CHO cells (mock).SpSLC9C1 in flagella and heads was probed with the anti-SpSLC9C1 antibody SU2 (left panel) andSpSLC9C1-HA in CHO K1 cells was probed with an HA antibody (right panel, see also Supplementary Figure8).bImmunocytochemical analysis of sperm stained with SU2 (left) and pre-immune serum control (right). Upper panels: bright-field (DIC) microscopy. Lower panels: overlay of DIC and fluorescence images (SpSLC9C1, green; nucleus stained with DAPI, blue). Scale bars represent 10 µm An acid-load experiment using control CHO cells [41] (Supplementary Figure 6a ) revealed endogenous amiloride-sensitive Na + /H + exchange; however, this exchange does not interfere with voltage-gated Sp SLC9C1 activity (Supplementary Figure 6b, c ): the voltage dependence of Sp SLC9C1 was similar in the absence and presence of amiloride (500 μM). In principle, Sp SLC9C1 could exhibit resting activity at depolarized voltages, similar to CNG channels that have been shown to have a non-zero open probability in the absence of ligand [42] . We tried to estimate the resting activity of Sp SLC9C1 at depolarized voltages (−30 mV) in the presence of amiloride (500 µM) by exchanging solutions from symmetrical with respect to Na + and H + to asymmetrical. 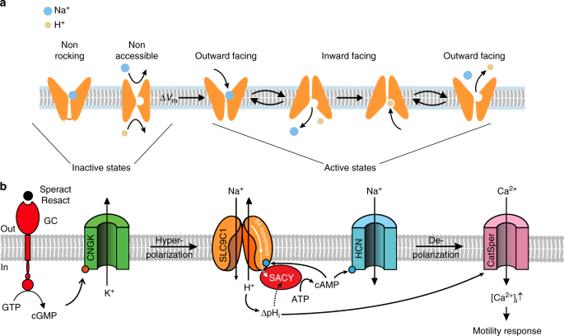Fig. 7 Models of SLC9C1 gating by voltage and cAMP.aCartoon depicting thatSpSLC9C1 is active only when the voltage enables its activity. The VSD could gate exchange activity by providing access for ions to their binding sites either by removing a physical gate or by enhancing the binding affinity for uploading (non-accessible). Alternatively, in the resting state, ions have access to their binding sites, but the rocking mechanism is locked (non-rocking); voltage unlocks the rocking motion and thus allows switching between outward- and inward facing conformations.bChemotactic signaling pathway in sea urchin sperm. Chemoattractant binding results in cGMP production and CNGK channel opening. The subsequent hyperpolarization activates SLC9C1. Alkalinization and cAMP production cooperate to open the CatSper channel. The intimate interaction between the exchanger and the soluble adenylate cyclase SACY is illustrated Under these conditions, we observed no significant change in pH i (Supplementary Figure 7a , n = 5 experiments). A subsequent voltage step to −100 mV again elicited Sp SLC9C1 activity. The normalized and background corrected resting activity under these conditions was 4.3 × 10 −3 ± 2.0 × 10 −2 (range −2.5 × 10 −2 to 3.1 × 10 −2 ). Therefore, we believe that it is safe to estimate that the resting activity is below 3% of its maximum value (Supplementary Figure 7b ). Cyclic AMP modulates gating currents and exchange activity Although the CNBD domain of Sp SLC9C1 is suggestive, several ion channels and protein kinase A (PKA) orthologues that carry a CNBD domain are, in fact, not gated or activated by cyclic nucleotides [5] , [43] , [44] . Therefore, we examined the action of cyclic nucleotides on gating currents and Na + /H + exchange (Figs. 2 and 4 ). Fig. 4 Modulation of Sp SLC9C1 activity by cAMP. a Action of 1 mM cAMP in the pipette solution on the voltage dependence of Sp SLC9C1 ( V 1/2 = −53.4 mV). ([Na + ] o 0 mM; [Na + ] i 14 mM; pH i = 7.2; pH o = 7.4). b Normalized Δ R values were plotted against V m to yield the V 1/2 values by a fit with the Boltzmann equation (w/o cNMP: V 1/2 = −70.9 ± 2.5 mV, s = 3.3 ± 0.9 mV, n = 7; cAMP: V 1/2 = −56.8 ± 2.7 mV, s = 4.6 ± 1.5 mV, n = 7; cGMP: V 1/2 = −67.8 ± 5.4 mV, s = 2.8 ± 1.0 mV, n = 9). c Flash photolysis of caged cAMP enhanced Sp SLC9C1 activity at a holding voltage of −63 mV and saturated after 3–4 flashes, same conditions as in a . d Normalized Δ R values were plotted against the number of flashes. Black circles show values from c . Decreasing the light energy of the flash, saturation of Sp SLC9C1 activity required 5–6 flashes (white circles). e The shift of V 1/2 and s values evoked by flash photolysis were similar to those using cAMP in the pipette (black triangles: V 1/2 = −55.3 ± 5.1 mV, s = 5.0 ± 0.6 mV, n = 3; for comparison: w/o cNMP (black circles) and 1 mM cAMP (white circles). f Replacing the Arg1053 in the CNBD by Gln (R1053Q) maintained a wild-type-like V 1/2 in the absence of cNMP (−70.8 ± 4.8 mV, s = 3.6 ± 1.1 mV, n = 5), but strongly reduced the V 1/2 shift by cAMP (−69.5 ± 3.8 mV, s = 3.9 ± 1.2 mV, n = 6). Mean values are summarized in Table 1 Full size image Cyclic AMP (1 mM) in the pipette shifted the V ½ of gating currents by 20 mV to −74.4 ± 6.4 mV, whereas cGMP (1 mM) was much less effective (Fig. 2b ). The number of gating charges was similar in the absence and presence of cAMP or cGMP. Similarly, cAMP shifted the V ½ of gating-current activation of the VSD mutant R803Q by 21 mV to −96.8 ± 6.6 mV (Fig. 2c ; Table 1 ). When cNMP binding was disabled by replacing a key Arg with a neutral residue in the phosphate-binding cassette of the CNBD (R1053Q) [45] , [46] , [47] , charge movement in the absence of cAMP was not affected, but the cAMP-induced V ½ shift was abolished (Fig. 2d ). Finally, this V 1/2 shift was not affected by the R399A mutation in the exchanger domain (Fig. 2e ). This result demonstrates that binding of cAMP to the CNBD changes the VSD equilibrium. Next, we examined whether cyclic nucleotides control exchange activity (Fig. 4 ). With cAMP (1 mM) in the pipette, the V ½ of exchange activity was shifted by 15 mV to −56.8 ± 2.7 mV (Fig. 4a, b ; Table 1 ). Again, cGMP was much less effective (Fig. 4b ). To compare Na + /H + exchange without and with cAMP in the same cell, we rapidly photo-released cAMP from caged derivatives of cAMP (BCMCM-cAMP and BECMCM-cAMP) [48] . At −63 mV, reverse-mode activity produced only a small acidification. Photo-release of cAMP instantaneously stimulated exchange activity (Fig. 4c ). The action of cAMP saturated after a few flashes (Fig. 4d ). At higher light intensity, the number of flashes required to saturate the response was lower (Fig. 4d ). The V ½ and s of activation after photolysis (−55.3 ± 5.1 mV and 5.0 ± 0.6 mV ( n = 3), respectively) was similar to that recorded in the presence of cAMP in the pipette (Fig. 4e ). Finally, in the R1053Q mutant with disabled CNBD, the activation of Na + /H + exchange by voltage was not altered, but the V ½ shift by cAMP was abolished (Fig. 4f ). These results demonstrate that binding of cAMP to the CNBD modulates Na + /H + exchange by shifting the voltage dependence of activation. Sp SLC9C1 mediates the chemoattractant-induced alkalinization Stimulation of sperm from S. purpuratus and Arbacia punctulata with chemoattractant peptides evokes a transient hyperpolarization and a rapid alkalinization [9] , [14] , [15] , [16] , [17] , [18] , [49] , [50] , [51] . When the hyperpolarization was abolished, the alkalinization was abolished as well [17] . We studied whether this alkalinization is caused by Na + /H + exchange via Sp SLC9C1. Using a rapid-mixing technique, we followed kinetically H + efflux and Na + influx in S. purpuratus sperm. Changes in pH i and intracellular Na + concentration ([Na + ] i ) were measured using BCECF and Asante Natrium Green-2, respectively. Stimulation with the chemoattractant speract elevated pH i and [Na + ] i with a similar dose dependence, time course, and latency (Fig. 5a, b ). The relation between the latencies of Na + and pH i responses was linear (slope of 1) over two orders of speract concentrations (Fig. 5b inset), indicating that H + efflux and Na + influx are mechanistically coupled. To investigate whether Sp SLC9C1 mediates Na + /H + exchange in sea urchin sperm, we studied the cAMP dependence of ion exchange by loading sperm with DEACM-caged cAMP [52] . We studied the action of cAMP photorelease on the resact-evoked pH i responses (Fig. 5c ). For all speract concentrations, the pH i response was faster and larger when cAMP was released (Fig. 5c ). The exchange activity was analyzed by plotting the maximal slope of the pH i change in the absence (black) or presence (red) of cAMP uncaging (Fig. 5d ). When cAMP was released, exchange activity was enhanced at all speract concentrations (Fig. 5d ). As control, we studied speract-evoked voltage signals with and without uncaging cAMP. Voltage responses were not affected by uncaging cAMP (Fig. 5e ), demonstrating that the enhanced exchanger activity is not due to a larger hyperpolarization. Fig. 5 Sodium and proton fluxes in S. pupuratus sperm. a Speract-induced changes in fluorescence ratio (Δ R / R ) indicating Na + influx (ANG2, black) or proton efflux (pH i ) (BCECF, red); signals were scaled and superimposed. Speract concentrations are shown on the right. b Mean latency ± SD ( n = 7) of pH i and Na + signal plotted vs. speract concentration. Inset: latency of pH i and Na + signal at different speract concentrations (10 pM black circles; 100 pM white circles; and 1 nM triangles). The line represents the identity function ( n = 7). c Speract-induced alkalinization monitored by pHrodo Red fluorescence in the absence (black trace) or presence (red trace) of release of cAMP from DEACM-caged cAMP with a continuously pulsing UV-LED. UV light was applied during the entire recording time. d The maximal slope of the pHrodo Red time course was plotted vs. speract concentration in the absence (black) and presence (red) of cAMP released from DEACM-caged cAMP ( n = 3). e Voltage recordings during speract stimulation (1 nM) in the absence (black) or presence (red) of cAMP released from DEACM-caged cAMP Full size image Blockers of SLC9A exchangers, including amiloride, failed to inhibit Sp SLC9C1 in heterologous systems. Similarly, in sea urchin sperm, the speract-induced pH i signals were largely unaffected by amiloride (500 µM, Supplementary Figure 5 e, f). In western blots of flagellar membranes, a polyclonal antibody raised against Sp SLC9C1 recognized three proteins with apparent M w of 132, 137, and 146 kDa similar to the M w of 146.6 kDa predicted for Sp SLC91 and to the apparent M w of HA-tagged Sp SLC9C1 in CHO cells (Fig. 6a and Supplementary Figure 8 ). The two prominent protein bands at higher M w might represent dimers and tetramers. Sp SLC9C1 was less abundant in head compared to flagellar preparations (Fig. 6a and Supplementary Figure 8 ). Multiple bands may indicate heterogeneous posttranslational modification. Finally, in immunocytochemistry, the antibody stained the flagellum and also partially the head (Fig. 6b ). These results confirm the presence of Sp SLC9C1 in Strongylocentrotus purpuratus sperm [53] . Altogether these experiments suggest that Sp SLC9C1 mediates the chemoattractant-induced alkalinization. Fig. 6 Analysis of Sp SLC9C1 expression in sea urchin sperm. a Representative western blot using protein lysates from flagella and heads of S. purpuratus sperm, from CHO cells heterologously expressing HA-tagged Sp SLC9C1 ( Sp SLC9C1-HA), and from non-transfected CHO cells (mock). Sp SLC9C1 in flagella and heads was probed with the anti- Sp SLC9C1 antibody SU2 (left panel) and Sp SLC9C1-HA in CHO K1 cells was probed with an HA antibody (right panel, see also Supplementary Figure 8 ). b Immunocytochemical analysis of sperm stained with SU2 (left) and pre-immune serum control (right). Upper panels: bright-field (DIC) microscopy. Lower panels: overlay of DIC and fluorescence images ( Sp SLC9C1, green; nucleus stained with DAPI, blue). Scale bars represent 10 µm Full size image Slc9 genes encode a large family of cation/proton-coupled antiporters, which fall into three subgroups: classical Na + /H + exchangers of the SLC9A (also referred to as NHE) subtype, the SLC9B (NHA) subtype, and SLC9C (sNHE) subtype. The SLC9A subfamily has been studied extensively, whereas, apart from gene-inactivation studies, little is known about SLC9B and SLC9C (SLC9B1 [54] ; SLC9C1 [2] ). Here, 15 years after the discovery of the SLC9C1 gene, we demonstrate that Sp SLC9C1 represents an electroneutral Na + /H + exchanger with a truly remarkable activation mechanism. Like voltage-activated ion channels, Sp SLC9C1 is gated by movement of a voltage sensor; this movement is controlled by cAMP binding to a C-terminal cyclic nucleotide-binding domain. The VSD of Sp SLC9C1 harbors seven positively charged amino acids in the S4 motif. Assuming a simple two-state Boltzmann mechanism of VSD movement, we estimate for Sp SLC9C1 activation an effective valence or gating charge g q of 3.1 e 0, which is similar to that of Shaker K + channels ( g q values of 2.5 e 0 per subunit [55] or 12–13 e 0 per tetrameric channel [56] ). Thus, the number of charges transported across the membrane during gating is similar in Shaker channels and Sp SLC9C1. For the only other non-channel VSD in a lipid phosphatase of Ciona intestinalis sperm, g q values are 1–1.6 e 0 [57] , [58] . How is Sp SLC9C1 activity controlled by the VSD? In general, solute carriers undergo cycles of conformational changes for upload and release of substrates on opposite sides of the membrane—a mechanism known as alternating access model [59] or rocking mechanism. A defining feature of this model is that ions or substrates themselves gate the conformational change and that solutes passively redistribute in response to extra- or intracellular changes in substrate concentrations. By contrast, in Sp SLC9C1, movement of a channel-like VSD couples membrane voltage to ion exchange. We envisage two different gating mechanisms. In one model, at resting voltage, either ions cannot reach the binding site, because access is obstructed by a physical gate, or ions cannot be uploaded, because the binding affinity is low (non-accessible, Fig. 7a ). Hyperpolarization opens the gate or enhances the binding affinity. Alternatively, at rest, ions can access and be uploaded to the binding site, but the rocking motion is blocked (non-rocking, Fig. 7a ) and hyperpolarization enables this exchange motion. These mechanisms are summarized by an extended kinetic scheme of exchange activity [60] (Supplementary Figure 7c ). A corollary of this scheme is that the exchanger—like ion channels—may have a small basal activity. Fig. 7 Models of SLC9C1 gating by voltage and cAMP. a Cartoon depicting that Sp SLC9C1 is active only when the voltage enables its activity. The VSD could gate exchange activity by providing access for ions to their binding sites either by removing a physical gate or by enhancing the binding affinity for uploading (non-accessible). Alternatively, in the resting state, ions have access to their binding sites, but the rocking mechanism is locked (non-rocking); voltage unlocks the rocking motion and thus allows switching between outward- and inward facing conformations. b Chemotactic signaling pathway in sea urchin sperm. Chemoattractant binding results in cGMP production and CNGK channel opening. The subsequent hyperpolarization activates SLC9C1. Alkalinization and cAMP production cooperate to open the CatSper channel. The intimate interaction between the exchanger and the soluble adenylate cyclase SACY is illustrated Full size image During their lifetime, sperm are exposed to vastly different aqueous conditions and compartments, involving large changes in external pH o and [Na + ] o [61] . Gating of Na + /H + exchange by voltage implies that extracellular changes are not relayed to the cytosol, unless triggered by a change in voltage that initiates rapid substrate redistribution. This mechanism might safeguard sperm from their environment and is functionally important for rapid periodic stimulation, while navigating in a chemical gradient. In conclusion, SLC9C1 represents a rapidly responding signaling molecule rather than a transporter for housekeeping pH i homeostasis. This study also provides insight into the puzzling function of cAMP in sperm from marine invertebrates. Whereas the role of cGMP in chemotactic signaling has been established [62] , the physiological function of cAMP remains elusive (Fig. 7b ). With the regulation of Sp SLC9C1 activity by cAMP, previously unexplained observations fall into place. For example, the hyperpolarization-evoked alkalinization persists for several tens of seconds [9] , whereas the hyperpolarization succumbs within a second [50] . The cAMP-induced V ½ shift of Sp SLC9C1 activation from −72 to −55 mV implies that Na + /H + exchange now also operates and maintains alkaline pH i near resting V m (about −50 mV). The alkalinization primes CatSper channels to open and promotes Ca 2+ entry [9] . Thus, cAMP, by maintaining alkaline pH i , keeps CatSper channels primed. This mechanism enables CatSper to translate rapid periodic V m changes into periodic Ca 2+ signals while sperm swim on a periodic path in a chemical gradient [9] . How is cAMP synthesis controlled? A soluble adenylate cyclase (SACY) is the predominant source for cAMP in sperm [63] , [64] . There is evidence for a direct physical interaction between SLC9C1 and sAC [12] , [64] . What is the functional role of this interaction? Whereas in many species, activity of SACY is controlled by bicarbonate and Ca 2+ [65] , [66] , [67] , circumstantial evidence indicates that cAMP synthesis in sea urchin sperm might be directly or indirectly regulated by membrane voltage [49] , or by pH i [68] , or some other mechanism. We speculate that Sp SLC9C1 confers voltage sensitivity to SACY either directly via its VSD or indirectly via alkalinization (Fig. 7b ). In turn, cAMP regulates Na + /H + exchange (Fig. 7b ). Future studies need to address this potential reciprocal control of SLC9C1 and SACY in sperm of sea urchin, vertebrates, and mammals. Functionally important amino-acid residues in the exchange domain are conserved between archaeal Na + /H + exchangers, mammalian SLC9A members, and Sp SLC9C1 (Supplementary Figure 1 ). Moreover, the VSD and CNBD domains of Sp SLC9C1 are functional and feature all structural hallmarks of the respective domains in voltage-gated ion channels and cyclic nucleotide-sensitive proteins (Fig. 1 and Supplementary Figure 1 ). In comparison, mammalian SLC9C1 members display several variations of functionally important residues. For example, the ND motif, which is part of the cation-binding site and which is characteristic of 1:1 Na + /H + exchangers, is replaced by a TS motif in mammalian SLC9C1 members. This might be a clue that mammalian SLC9C1 proteins acquired different functions. Finally, three of the four N-terminally located Arg or Lys residues in the S4 motif of Sp SLC9C1 are missing in mouse and human orthologues (Fig. 1c ), suggesting that voltage activation of mammalian SLC9C1 proteins may be different. Thus, our work provides a technical and conceptual blueprint for future studies of mammalian SLC9C1 orthologues. Strongylocentrotus purpuratus sperm samples Collection of dry sperm was described previously [62] . In brief, 0.2–0.5 ml of 0.5 M KCl was injected into the sea urchin cavity to induce spawning. Spawned sperm (dry sperm) were collected using a Pasteur pipette and stored on ice. Measurement of [Na + ] i , pH i , and V m in S. purpuratus sperm We measured speract-induced changes in [Na + ] i , pH i , and V m by loading sperm samples with the corresponding dye (Asante Natrium Green 2/ANG2, TEFLabs, Austin, USA; BCECF-AM and pHrodo Red-AM, both from Molecular Probes, Eugene, USA; and di-4-AN(F)EP(F)PTEA [69] (kind gift of Dr. L. Loew) in a rapid mixing device (SFM-400, BioLogic, Claix, France) [62] . Dry sperm was suspended 1:6 (v/v) in Artificial Sea Water (ASW) containing (in mM); NaCl 423, CaCl 2 9.27, KCl 9, MgCl 2 22.94, MgSO 4 25.5, EDTA 0.1, HEPES 10 at pH 7.8, and the respective dye (18 °C). Loading concentrations and times were: ANG2: 10 µM for 60 min (0.5% w/v Pluronic F127, Molecular Probes); BCECF-AM: 10 µM for 10 min; pHrodo Red-AM: 16 µM for 30 min (0.5% Pluronic F127); di-4-AN(F)EP(F)PTEA: 25 µM for 5 min (0.5% Pluronic F127). After 1:20 (v/v) dilution in ASW, sperm were allowed to equilibrate for 5 min. Subsequently, sperm were mixed 1:1 (v/v) with speract in ASW. ANG2 signals in sperm were recorded at a flow rate of 1.3 ml s −1 . BCECF and pHrodo Red signals were recorded at flow rates of 1.3 ml s −1 (Fig. 5a ) or 4 ml s −1 (Fig. 5c ). di-4-AN(F)EP(F)PTEA signals were recorded at a flow rate of 4 ml s −1 . Fluorescence was excited by pulsed LED light (SpectraX Light Engine, Lumencor, Beaverton, USA or M490L3, Thorlabs, Newton, USA) with a frequency of 10 kHz or by high power LEDs (Thorlabs) with frequencies up to 80 kHz. Emission was recorded by photomultiplier modules (H9656-20 and C7169, Hamamatsu Photonics, Japan). The signal was amplified and filtered by a lock-in amplifier (7230 DualPhase, Ametek, Paoli, USA). Data acquisition was performed with a data acquisition pad (PCI-6221, National Instruments, Austin, USA) and Biokine Software v.4.49 (BioLogic). For [Na + ] i recordings, excitation light passed a 485/25 nm filter (AHF, Tübingen, Germany). The emitted fluorescence passed a 536/40 nm filter (Semrock, Rochester, USA). For BCECF recordings, excitation light passed a 452/45 nm filter (Semrock). BCECF fluorescence was recorded in dual-emission mode using Brightline 494/20 nm and 540/15 nm filters (Semrock). The pH i signals represent the ratio of F 494 / F 540 . They are the average of at least two recordings and are depicted as the percent change in ratio (Δ R / R ) with respect to the first 10–20 data points after mixing. For pHrodo Red recordings, excitation and emission were at 572/15 and 628/40 nm, respectively. For V m recordings, excitation light passed a 513/18 nm filter (Semrock); di-4-AN(F)EP(F)PTEA fluorescence was recorded in dual emission mode using Brightline 549/15 and 705/72 nm filters (Semrock). The V m signals (ratio F 549 / F 705 ( R ); average of at least four recordings) are depicted as the percent change in ratio (Δ R / R ) with respect to the first 10 data points. The baseline control (ASW) was subtracted from the speract-induced signals. To manipulate cAMP in sperm during chemoattractant stimulation, sperm were incubated with 30 µM DEACM-caged cAMP for 30–60 min. Uncaging was performed in the stopped-flow cuvette by a 360 nm LED (Thorlabs) with 58 kHz. Generation of a polyclonal anti- Sp SLC9C1 antibody Peptides comprising amino acids (aa) 574–591 (EFADMMEEARLRMLKAEK), aa 857–871 (MVDNKKILRELKHIS), aa 937–957 (KMKRLMNAPSSIPPPPPENLL), and aa 1111–1126 (GWTQEKVKLHLERGYL) were synthesized and coupled to BSA via a cysteine that was introduced at the N terminus of peptides. Rabbit antibodies directed against a mixture of these peptides, resulted in two polyclonal antibodies SU1 and SU2. The Sp SLC9C1 antibody was purified from antisera by affinity purification using the four peptides. All steps for antibody production were performed by Davids Biotechnology, Regensburg, Germany. Preparation of heads and flagella from S. purpuratus Sperm flagella and heads were separated as described [9] with one modification: instead of shearing with a 24-G needle, the sperm suspension was sheared 20 times by centrifugation for 30 s at 75 × g and 4 °C through the net of a 40-µm cell strainer (BD Biosciences). Cell lines CHO-K1 cells were obtained from European Collection of Authenticated Cell Cultures (ECACC, catalog number 85051005). Mycoplasma tests were carried out regularly, once a year. The results of the mycoplasma tests are available upon request. Western blotting Sperm flagella and heads from S. purpuratus , CHO K1 cells stably expressing HA-tagged Sp SLC9C1 ( Sp SLC9C1-HA), and CHO K1 control cells (mock) were lysed by sonification in a hypotonic buffer containing 10 mM Hepes/NaOH, pH 7.4, 2 mM EDTA, and protease inhibitor mixture mPIC (Sigma Aldrich, St. Louis, USA). The suspension was centrifuged for 10 min at 500 × g . The supernatant was used for Western blotting. Twenty µg protein per lane were separated by SDS-PAGE using a precast NuPage Novex 7% Tris-Acetat Protein Gel (Thermo Fisher Scientific, Waltham, USA). The samples were heated for 5 min at 95 °C prior to separation. Protein Marker VI (AppliChem, Darmstadt, Germany) and HiMark Pre-Stained Protein Standard (Thermo Fisher Scientific) were used as molecular weight markers. Proteins were transferred onto an Immobilon FL PVDF membrane (Merck Millipore, Darmstadt, Germany), probed with antibodies, and analyzed using the Odyssey Imaging System (LI-COR, Bad Homburg, Germany). All figure panels were taken from the same western blot. Figures were prepared using CorelDrawX6 and Photo-PaintX6 software (both from Corel Corporation). Primary antibodies were: Sp SLC9C1-SU2 (1:3000), rat-anti-HA (1:3000; Roche Applied Science catalog no. 11867431001, Penzberg, Germany). Secondary antibodies were as follows: IRDye680 and IR800 antibodies (LI-COR, 1:25,000). Cloning of S0p SLC9C1 Four sets of primer pairs, designed on the annotated sequence for the Strongylocentrotus purpuratus sperm-specific sodium proton exchanger, NM_001098457, were used to obtain the full-length sequence by PCR amplification on a Strongylocentrotus purpuratus testis library. Primers C0600, C0601, C0602, and C0603 were used to amplify the 5′ part of the sequence (bp 1 to 1444) by to rounds of PCR. Primer C0600 introduces a BamHI site followed by a perfect Kozak sequence [70] preceding the start codon. Primers C0601 and C0602 destroy the internal BamHI site at position 624 by a silent mutation. Primer C0603 introduces an EcoRI site. Primers C0604 and C0605 were used to amplify bases 1432 to 2734. Primer C0604 introduces a EcoRI site, primer C0605 introduces a XhoI site by silent mutation. The 3′ part (bp 2723 to 3975) was amplified with primers C0610, C0606, C0607 and C0608 in two rounds of PCR. Primers C0606 and C0607 destroy the internal XhoI site at position 3361 by a silent mutation. Primer C0610 introduces a XhoI site. Primer C0608 adds a sequence for an HA-tag to the 3′ end, followed by a stop codon and an XbaI site. The primer sequences were: ACAGGATCCACCATGAAGAAGAGAGTCGTGAAATTG (C0600), CGACGGGATCTGTCGCACTCATG (C0601), CATGAGTGCGACAGATCCCGTCG (C0602), CCAGAATTCTCAGTAGAGTCTGGATGG (C0603), CTGAGAATTCTGGGCATGAGTGACATC (C0604), TCTCTCGAGAGTGGTTGAGAATGGTG (C0605), ACTCTCGAGAGACTATCCATGAACTCC (C0610) GCCACGCTCAAGATGTAACTTCAC (C0606), GTGAAGTTACATCTTGAGCGTGGC (C0607), and TCTTCTAGATTAGGCGTAGTCGGGCACGTCGTAGGGGTAAACGTTGACCCTAGGGGCC (C0608). All three resulting PCR fragments were cloned together into vector pcDNA3.1(+) (Invitrogen, Carlsbad, USA) to obtain the full-length clone. Generation of stable CHO cell lines of Sp SLC9C1 and h Hv1 CHO K1 cells were electroporated with pc3 sNHE-HA or with pc3 h Hv1 using the Neon 100 Kit (Invitrogen, Carlsbad, USA) and a MicroPorator (Digital Bio) according to the manufacturer’s protocol (3 × 1650 mV pulses with a 10-ms pulse width). Cells were transferred into complete medium composed of F12 plus GlutaMAX (Invitrogen) and 10% fetal bovine serum (Biochrom, Berlin, Germany). To select monoclonal cells stably expressing Sp SLC9C1 or h Hv1, the antibiotic G418 (1200 mg ml −1 ; Invitrogen) was added to the cell culture medium 24 h after the electroporation. Monoclonal cell lines were identified by immunocytochemistry using a rat-anti-HA antibody (Roche Applied Science) or by electrophysiological recordings. Immunocytochemistry Sperm samples were stained as previously described [9] . Antibodies were diluted 1:400 ( Sp SLC9C1-SU1) and 1:750 ( Sp SLC9C1-SU2) in 0.1 M phosphate buffer (pH 7.4) in the presence of 0.5% Triton X-100 and 5% chemiblocker (Millipore). Primary antibodies were incubated overnight at 4 °C and visualized by goat-anti-rabbit A488 (1:500, 20 min incubation at RT, ThermoFisher Scientific A-11034, Rockford, USA). In CHO cells, Sp SLC9C1-HA was probed by a rat-anti-HA antibody (1:1000, 1 h incubation at RT, Roche Applied Science) and visualized by goat-anti-rat A488 (1:400, 20 min incubation at RT, ThermoFisher Scientific A-11006). Membrane sheet preparations were obtained by sonification (0.1 s, 5%, Vibracell, Sonics & Materials, Newtown, USA) of CHO cells plated on poly-lysine (0.1 mg ml −1 , Sigma Aldrich) coated glass coverslips (Marienfeld-Superior, Lauda-Königshofen, Germany) in HEPES-buffered solution (1 mM DTT, 0.2% mPIC v/v). As marker for outer plasma membrane, CHO cells were additionally transfected with membrane-bound CAAX-RFP protein. For labeling the ER, a calnexin antibody was used (mouse-anti-calnexin, 1:500, Abcam ab31290, Cambridge, UK). Solutions for patch-clamp recordings Intracellular Solution (IS, in mM): NaCl 10, KAsp 130, EGTA 10, MgCl 2 1, Na 2 ATP 2, HEPES 1, adjusted to pH 7.2 with KOH (3 M). Extracellular Solution (ES, in mM): NaCl 140, KCl 5.4, MgCl 2 1, CaCl 2 1.8, HEPES 5, Glucose 10, adjusted to pH 7.4 with NaOH (1 M). ES-NMDG, NaCl substituted for N -methyl- d -glucamine (NMDG) and was adjusted to pH 7.4 with HCl. Single-cell fluorimetry We recorded in the whole-cell configuration changes in pH i from CHO cells expressing Sp SLC91 (wt), either stably expressed or using transient expression, or the respective Sp SLC91 mutants, using transient expression. For the determination of the voltage dependence of transport activity, we co-expressed h Hv1 with Sp SLC91 (wt), or the mutants Sp SLC9C1-R1053Q or Sp SLC9C1-R803Q. Cells were loaded with BCECF (10 µM) via the pipette and were excited with a Photon Technology International DeltaRam X TM monochromator (PTI, New Jersey, USA). BCECF fluorescence was recorded in dual-excitation mode at 440 ± 6.25 nm and at 480 ± 6.25 nm with 5-Hz frequency (100 ms nm −1 ). Emitted light passed a dichroic mirror (500 nm LP) and a 525/15 nm filter (Semrock) and was detected by a photomultiplier system (Model 814, PTI). The pH i signals represent the ratio of F 480 / F 440 . We used a gravity-driven perfusion system. Temperature of ES and ES-NMDG solutions was set to 28 °C by a HPT-2 Heated Perfusion Tube (ALA Scientific Instruments Inc. St. Farmingdale, USA). For analysis of V ½ and slope (s) of Sp SLC9C1 activity, the initial slope of the Δ R signal was fitted by linear regression. The resulting slopes were plotted against voltage and were fitted to a Boltzmann equation \(\Delta R\left( V \right) = \Delta R_{{\mathrm{max}}}/\left( {1 + \exp (V - V_{1/2})/s} \right)\) with s = ( kT) /( q g × q e ). k = 1.38 × 10 −23 J K −1 , T = 301.15 K (28 °C), and q e = 1.6 × 10 −19 As. V ½ is the potential where Δ R ( V ) = Δ R max /2. To determine mean Δ R values across data sets, we normalized each dataset to the corresponding parameters of the Boltzmann fit. For experiments with caged compounds, we loaded cells with membrane-permeant caged cyclic BECMCM-caged cAMP (10 µM) for 30 min prior to measurement and included also 100 µM BCMCM-caged cAMP in the pipette solution. Flash photolysis was achieved with short UV pulses (~1 ms) via a Xenon flash lamp System (JML-C2, Rapp OptoElectronic, Hamburg, Germany); light was passed through a UV filter (UV-2 250-375, Rapp OptoElectronic). Light energy was adjusted through the loading voltage of the lamp’s capacitor and by neutral density gray filters (300 V, OD1 in Supplementary Figure 3a ; 200 V, OD0.4 in Supplementary Figure 3b ). The calibration procedure for BCECF fluorescence to yield pH i by the pseudo-null-point method [33] was described previously [9] . Briefly, wild-type or Sp SLC9C1 expressing CHO cells seated on glass coverslips were loaded with 10 µM BCECF-AM for 10 min. Coverslips were placed into a home-built perfusion chamber on an Olympus cell R single-cell imaging system. Fluorescence at 540 nm was recorded ratiometrically by alternating excitation using 430/20 nm and 470–490 nm filters, yielding R = F480/F430. The pH i pseudo-null-point solutions contained defined concentrations of weak acid (propionic acid) and weak base (ammonium chloride) in ES solution. In the neutral form, weak acids and bases permeate the plasma membrane resulting in a transient change in pH i . The extent and direction of the change in pH i can be predicted by \({\mathrm{pH}}_{\mathrm{null}} = {\mathrm{pH}}_{\mathrm{o}} - 0.5\hskip 3pt{\mathrm{log}}[A]/[B]\) , wherein [ A ] refers to an acid and [ B ] to a base. The concentrations of propionic acid (5 mM) and ammonium chloride (0.05, 0.32, 1.99, 12.56, 79.25 mM) yielded pH null solutions of 6.4, 6.8, 7.2, 7.6, and 8.0, respectively. To prevent side effects due to osmolarity issues, the NaCl concentration of the ES solution was respectively adjusted (134.95, 134.68, 133.01, 123.44, 55.75 mM for pH null of 6.4, 6.8, 7.2, 7.6, and 8.0). Gating currents We recorded gating currents in CHO cells expressing Sp SLC9C1 (wt), Sp SLC9C1-R1053Q, SpSLC9C1-R399A, or Sp SLC9C1-R803Q in ES at 28 °C. Online P/N leak subtraction was performed with four pre-pulses (P/4) opposite to pulse polarity to subtract linear currents due to leakage or capacitive artifacts (Clampex V1.10.2.0.12, MDS Analytical Technologies). Voltage steps ranging from +15 to −155 mV in steps of 10 mV were applied. Off-gating currents were integrated over time to yield net charges ( Q ). To quantify the voltage dependence of charge movement, we fitted Q / V curves to a Boltzmann equation, defined as \(Q\left( V \right) = 1/\left( {1 + \exp \left( {V - V_{1/2}} \right)/s} \right)\) with s = ( kT )/( q g × q e ). Mean gating charges ( Q / Q max ) were determined by normalizing each data set to the corresponding parameters of the Boltzmann fit. For the Sp SLC9C1-R399A mutant, not all gating - current recordings were performed with the same voltage protocol. The number of charges ( q g ) involved in the gating process was determined from q g = ( kT )/( s × q e ). Data availability The data that support the findings of this study are available from the corresponding authors upon request.